The IncP-1 plasmid backbone adapts to different host bacterial species and evolves through homologous recombination Plasmids are important members of the bacterial mobile gene pool, and are among the most important contributors to horizontal gene transfer between bacteria. They typically harbour a wide spectrum of host beneficial traits, such as antibiotic resistance, inserted into their backbones. Although these inserted elements have drawn considerable interest, evolutionary information about the plasmid backbones, which encode plasmid related traits, is sparse. Here we analyse 25 complete backbone genomes from the broad-host-range IncP-1 plasmid family. Phylogenetic analysis reveals seven clades, in which two plasmids that we isolated from a marine biofilm represent a novel clade. We also found that homologous recombination is a prominent feature of the plasmid backbone evolution. Analysis of genomic signatures indicates that the plasmids have adapted to different host bacterial species. Globally circulating IncP-1 plasmids hence contain mosaic structures of segments derived from several parental plasmids that have evolved in, and adapted to, different, phylogenetically very distant host bacterial species. The ability of prokaryotes to exchange genes by means of horizontal gene transfer (HGT) has far-reaching implications for our understanding of prokaryotic evolution [1] , [2] , [3] , [4] . One of the most important contributors to HGT is conjugative plasmids, which are self-replicating extra-chromosomal units that code for their own cell-to-cell conjugal transfer systems. The plasmid backbone, which contains genes encoding plasmid-related traits, such as replication control and conjugation functions, is usually loaded with accessory genes, such as antibiotic-resistance and heavy-metal-resistance genes. These are themselves often part of other mobile genetic elements (MGEs), such as transposons and integrons. Plasmids are important in bacterial evolution and in adaptation to environmental changes, because they may carry genes that are useful to the host bacterium. The resulting fitness of a plasmid can therefore be thought of as the sum of a 'selfish' component, including conjugative transfer, replication and various maintenance functions, and a component that confers advantages on the host cell, exemplified by antibiotic-resistance genes [5] . The development of antibiotic resistance in pathogenic bacteria is a serious and growing health concern. One particularly problematic development is the emergence of multiresistance; that is, bacteria becoming resistant to many, if not all, medically used antibiotics. Plasmids have an important role in the spread of antibiotic-resistance genes between bacteria and in the development of multiresistance [6] , [7] , [8] . Knowledge of the manner in which plasmids evolve is thus important if we are to better understand the fundamentals of prokaryotic evolution and the principles underlying the accumulation and spread of antibiotic resistance in bacterial communities. Research into IncW plasmids [9] and F plasmids [10] has suggested recombination, and that rare recombination events may be a driving force behind the creation of new plasmid families. The IncP-1 plasmid group has a broad host range and can be stably maintained in almost all Gram-negative bacteria. IncP-1 plasmids have also been demonstrated to conjugate to Gram-positive bacteria [11] and to yeast and eukaryotic cell lines [12] , [13] . A recent study using genomic signatures also suggested a broad host range of the IncP-1 plasmids [14] . Furthermore, they can also harbour a wide spectrum of antibiotic-resistance genes [7] . Five evolutionary clades have hitherto been described for IncP-1 plasmids: α-clade [15] , β-clade [16] , γ-clade [17] , [18] , δ-clade [17] and ɛ-clade [19] . Several previous studies of the evolution of these plasmids focus on differences in MGE incorporated into the backbone [20] , [21] , [22] . Incorporation and expelling of such elements occur more frequently than do changes in the core backbone, exemplified by plasmids with similar backbones, harbouring different transposons ( [15] , [20] , [23] ; and the present report), thus providing information on the relatively recent evolution of the plasmids. Long-term evolution, however, should preferably be based on 'deep characters', and analysis of the plasmid backbone may reveal important information on how these plasmids evolve and adapt to their hosts. Information about recombination of the IncP-1 plasmid backbone has hitherto been sparse, except in a few studies in which occasional recent recombination events were suggested [19] , [24] . It has been suggested that recent human activities, such as the use of wastewater treatment plants that mix bacteria from a large number of sources, would increase contacts between bacteria and therefore increase recombination between plasmids [7] . Furthermore, the increased mobility of people and goods would be expected to increase the worldwide spread of these plasmids. Isolation of similar plasmid backbone sequences from different parts of the world seems to support this hypothesis [19] . Here we analysed the complete backbone genomes of 25 IncP-1 plasmids, including two novel plasmids from the marine environment. We demonstrate that recombination is not only a recent phenomenon induced by human interference but also has been a continuous and prominent feature of the IncP-1 backbone evolution. Considering recombination, we describe a consensus phylogeny of the IncP-1 plasmids presenting a divergence into seven distinct clades. We also analysed plasmid DNA signatures and suggest that the IncP-1 plasmids have different host species histories, and that the plasmids have been temporarily isolated in different host bacteria for sufficiently long times for their genomic signatures to have been influenced. Plasmid backbone analysis We analysed the complete backbone DNA sequences of two novel IncP-1 plasmids, designated as pMCBF1 and pMCBF6, isolated from a marine biofilm [25] , and compared them with 23 previously described IncP-1 plasmids retrieved from GenBank (found through BLAST and literature searches). These include the IncP-1 plasmids that resulted from a recent thorough plasmid search [14] . Plasmids pMCBF1 (62,689 bp) and pMCBF6 (66,729 bp) presented identical backbones and differed only in their mercury-resistance transposons, the common backbone will hereafter be referred to as pMCBF1. Putative gene functions are shown in Tables 1 and 2 . 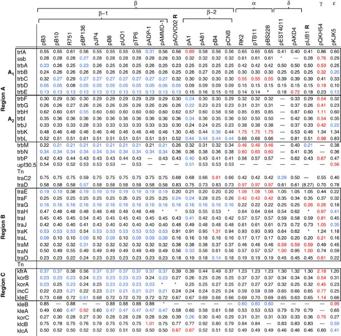Figure 1: Genetic distances between pMCBF1 and other fully sequenced IncP-1 plasmids. Genetic distances between each gene in pMCBF1 and the corresponding genes in the other 23 analysed plasmids. The plasmid(s) with the longest distance to pMCBF1 is marked in red and the plasmid(s) with the shortest distance is marked in blue for respective gene. Genes not present in specific plasmids are marked with '–' and genes that are at least partially present but not expressed as proteins, or proteins not annotated in GenBank are marked with '*'. Three genomic regions, A (further divided into two subregions A1and A2), B and C were identified as suitable targets for further phylogenetic and signature analysis as they were present in all plasmids. Table 1 Location and putative function of the predicted coding regions of pMCBF1. 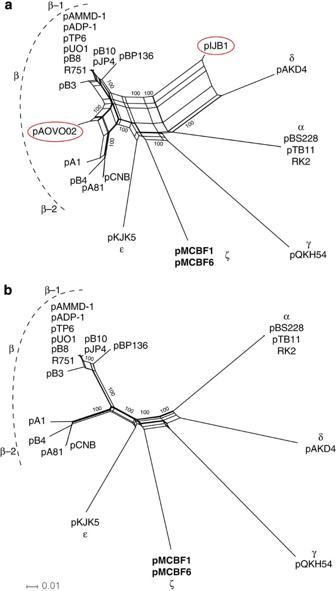Figure 2: Phylogenetic analysis of the IncP-1 plasmid backbone. (a) Phylogenetic network based on the concatenated backbone regions A, B and C of 25 IncP-1 plasmids. The network displays seven main clades, including a novel clade containing the two newly sequenced plasmids pMCBF1 (in bold) and two sub-clades, β-1 and β-2, of the previously described β-clade. The putative recent recombinant plasmids pIJB1 and pAOVO02 are marked with red ellipses. (b) Phylogenetic network excluding the putative recent recombinant plasmids pIJB1 and pAOVO02. Full size table Table 2 Location and putative function of the predicted coding regions of transposon Tn5058 in pMCBF6. Full size table The genetic distance between the amino-acid (AA) sequence of each backbone gene in pMCBF1 and their corresponding genes in the 23 previously described IncP-1 plasmids was estimated by a maximum likelihood approach. The backbone gene content in the 25 plasmids differs significantly and only 24 homologues of the 41 backbone genes in pMCBF1 were present in all analysed plasmids ( Fig. 1 ). The AA similarity differed also widely with trbD being the most conserved gene. Among all 23 plasmids, plasmid pB4 presents the closest genetic distance to pMCBF1 in genes trbK , trbL , traG and traO , whereas pB4 genes traC2 and traK present the longest genetic distance. Similarly, the pKJK5 genes trbB , trbE , trbJ , traH , traJ , klcB and klcA presented the closest, and the two genes upf30.5 and kleB in the same plasmid presented the longest genetic distance to pMCBF1. Only plasmids pAKD4 and pQKH54 did not have any gene with the closest genetic distance to pMCBF1. Such alterations of relative genetic distances may be explained either by unequal nucleotide substitution rates or by an evolutionary history including homologous recombination (that is, the fact that the different genes in each plasmid backbone have different ancestries). Figure 1: Genetic distances between pMCBF1 and other fully sequenced IncP-1 plasmids. Genetic distances between each gene in pMCBF1 and the corresponding genes in the other 23 analysed plasmids. The plasmid(s) with the longest distance to pMCBF1 is marked in red and the plasmid(s) with the shortest distance is marked in blue for respective gene. Genes not present in specific plasmids are marked with '–' and genes that are at least partially present but not expressed as proteins, or proteins not annotated in GenBank are marked with '*'. Three genomic regions, A (further divided into two subregions A 1 and A 2 ), B and C were identified as suitable targets for further phylogenetic and signature analysis as they were present in all plasmids. Full size image To reconstruct their evolutionary history, it was necessary to base the phylogenetic analysis on backbone regions, which are conserved and present in all 25 plasmids. Three such relatively large regions were identified and here referred to as regions A, B and C ( Fig. 1 ). Region A was further divided into subregions A 1 and A 2 to decrease its size. Region A 1 contains the seven genes trfA , ssb , trbA , trbB , trbC , trbD and trbE . Although the AA sequences for the genes ssb and trbE in plasmid pEST4011 and pBS228, respectively, was not available because of 'truncation by insertion', the counterpart of the genes was still present, allowing it to be included for analysis. Region A 2 contains the seven genes trbF to trbL . Region B contains the 11 genes traE to traO , and region C contains the five genes kfrA , korB , korA , incC and kleE . The DNA sequences were aligned and gap regions were excluded before further analyses. The four regions were also concatenated and analysed as one large ( ∼ 19,000 nucleotides) segment. Plasmid pIJB1 was previously described as a recombinant [26] with a duplication of the genes trfA to trbE . In this study, we included the second duplicate in the analysis to analyse an intact A region. Phylogenetic analysis of the IncP-1 backbone A splits network ( Fig. 2a ) was initially constructed for 1,000 bootstrap replicates of the concatenated segments A 1 , A 2 , B and C of 24 IncP-1 plasmids (plasmid pEST4011 was excluded from the analysis as it lacks the genes in A 2 ). The network, which presents a combinatorial generalization of phylogenetic trees, presented a star-like topology with seven main clades. pMCBF1 formed a novel clade, hereafter called ζ. As visible in a previous study [26] , the β-clade [16] could be divided into two subclades, β-1 and β-2. Parallel edges in the phylogenetic network indicated, however, conflicting phylogenetic signals, possibly resulting from homologous recombination. In particular, in addition to plasmid pIJB1, plasmid pAOVO02 was a putative recombinant, not clustering to any of the above-described clades. A second network, excluding these two plasmids, was therefore constructed for comparison ( Fig. 2b ). Figure 2: Phylogenetic analysis of the IncP-1 plasmid backbone. ( a ) Phylogenetic network based on the concatenated backbone regions A, B and C of 25 IncP-1 plasmids. The network displays seven main clades, including a novel clade containing the two newly sequenced plasmids pMCBF1 (in bold) and two sub-clades, β-1 and β-2, of the previously described β-clade. The putative recent recombinant plasmids pIJB1 and pAOVO02 are marked with red ellipses. ( b ) Phylogenetic network excluding the putative recent recombinant plasmids pIJB1 and pAOVO02. Full size image Recombination analysis To investigate whether the conflicting phylogenetic signals are caused by homologous recombination or homoplasy, we initially used a statistical test, the φ -test, which was recently described to yield reliable results for diverged DNA sequences [27] . We analysed the complete concatenated segment, as well as three regions separately, to analyse the frequency and location of recombination crossovers (segments A 1 and A 2 were analysed as one segment A to decrease bias of multiple testing). To estimate the frequency of recombinant plasmids, we also divided the data set into six representative subgroups. These subgroups were selected on the basis of clade identity to analyse possible recombination events within the β-1 subclade, which harbour enough members to perform such analysis, and between the different clades. Because all three α-clade plasmids have identical backbone sequences, and because the ∑, γ, δ and ζ clades were represented by single backbones, it was impossible to investigate whether recombination had occurred within these clades. Consequently, the φ-test was applied on 28 data sets. After a Bonferroni correction for multiple tests, the significance level was set to P =0.05/28=0.002. 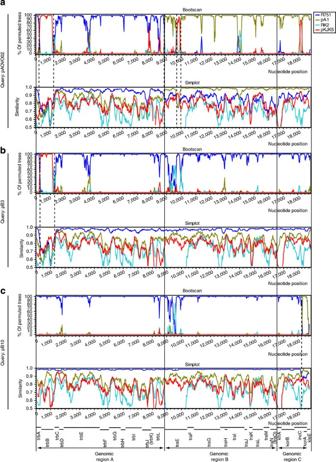Figure 3: Bootscan and SimPlot analysis. Analysis of the backbones of plasmids pAOVO02 (a), pB3 (b) and pB10 (c). Each coloured plot corresponds to a specific plasmid depicted in the colour shemes to the right. The bootscan plot demonstrates phylogenetic relationship to the reference strain, and the SimPlot demonstrates the genetic distances to the reference strain in different parts of the genome. Sudden alterations in bootstrap support, illustrated in the Bootscan plots, indicates recombination. Sequence similarity to the reference strains is represented in the similarity plots beneath the Bootscan plots. Obvious recombination crossovers are highlighted as dotted lines. High sequence similarity indicates recent recombination events. Low sequence similarity indicates ancient recombination events, alternatively recent recombination events involving unanalysed plasmids. The results ( Table 3 ) indicated strong statistical significance ( P <0.002) for recombination in the vast majority of the data sets. There was no statistically significant support for recombination crossovers within the three separate segments of the β-1 subclade plasmids or for the A-segment of the data set containing plasmids within subclade β-2 and pKJK5 or for the B-segment of the data set containing pQKH54, pMCBF1, RK2 and pTP6. However, there was high statistically significant support for recombination when the three concatenated segments were analysed, indicating that recombination crossovers are located between, but not necessarily within, the three investigated regions. Table 3 Statistical significance of recombination using the φ -statistics. Full size table To further explore and visualize putative recombination crossovers, we used the Bootscan method, which uses a sliding-window approach, in which a window of a fixed size is moved step-by-step through the sequence alignment. In each step a phylogenetic tree with bootstrap values for each clade is created. The putative recombinant is selected as the query, and the bootstrap support for each of the other plasmids being the one that clusters closest to the query is plotted. Recombination crossovers are indicated as sudden changes in bootstrap supports. Similarity plots were also constructed using a similar sliding-window approach, illustrating the DNA sequence similarity between the query and the other sequences. The Bootscan and similarity plots support recombination. One example is pAOVO02, which showed a pattern consistent with recombination between the putative parental plasmids R751, pA1 and pKJK5 ( Fig. 3a ). These were also supported as parental plasmids by the similarity plot, except for pKJK5, which showed a lesser similarity to pAOVO02 than the other two. Another example is pB3, which generally presented the closest evolutionary relationship to R751 ( Fig. 3b ) and a close sequence similarity (>95% on average). In a specific pB3 region, however, the Bootscan plot indicated a closer evolutionary relationship to pKJK5, even though the sequence similarity was only 68–88%. A similar alteration in bootstrap support was seen for pB10 ( Fig. 3c ), which mostly showed the closest relationship to R751 except in one region that was more related to plasmid pA1, supporting a previous suggestion about recombination in pB10 (ref. 24 ). The SimPlot also indicated a generally high similarity of >95% to R751 and a high similarity to pA1 in the specific region. Finally, additional SimPlot analyses were performed to investigate the ancestry of specific recombination fragments. For example, plasmids pB3 and pBP136 shared almost identical sequences with plasmid R751, except in a few regions in which the sequence similarity was significantly less ( Fig. 4a ). When pBP136 ( Fig. 4b ) and pB3 ( Fig. 4c ) were compared with all other plasmids studied here, none of them presented high similarities in these regions for plasmid pBP136 and only plasmid pAOVO02 showed a high similarity in the specific region of pB3. A BLAST search identified no sequence with close similarity to the three regions in pBP136. In summary, we find that the φ -test supports recombination between IncP-1 plasmids and Bootscan, and similarity plots further illustrate the recombination crossovers. Figure 3: Bootscan and SimPlot analysis. Analysis of the backbones of plasmids pAOVO02 ( a ), pB3 ( b ) and pB10 ( c ). Each coloured plot corresponds to a specific plasmid depicted in the colour shemes to the right. The bootscan plot demonstrates phylogenetic relationship to the reference strain, and the SimPlot demonstrates the genetic distances to the reference strain in different parts of the genome. Sudden alterations in bootstrap support, illustrated in the Bootscan plots, indicates recombination. Sequence similarity to the reference strains is represented in the similarity plots beneath the Bootscan plots. Obvious recombination crossovers are highlighted as dotted lines. High sequence similarity indicates recent recombination events. Low sequence similarity indicates ancient recombination events, alternatively recent recombination events involving unanalysed plasmids. 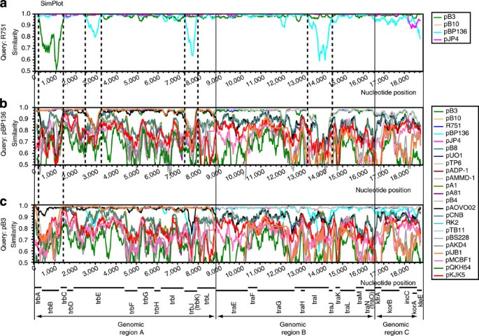Figure 4: SimPlot analysis. Similarity plots with plasmids R751, pBP136 and pB3 as reference plasmids. Each coloured plot corresponds to a specific plasmid depicted in the colour shemes to the right and demonstrates the genetic distances from each plasmid to the reference strain in different parts of the genome. The similarity plot of R751 (a) highlights one putative recombination event in plasmid pB3 and three putative recombination events in plasmid pBP136. The similarity plots of these two plasmids (b,c) demonstrate that none of the plasmids included in this study are donors of the recombinant regions in pBP136. Instead, other plasmids from clades that were not previously described were probably involved in these recombination events. Full size image Figure 4: SimPlot analysis. Similarity plots with plasmids R751, pBP136 and pB3 as reference plasmids. Each coloured plot corresponds to a specific plasmid depicted in the colour shemes to the right and demonstrates the genetic distances from each plasmid to the reference strain in different parts of the genome. The similarity plot of R751 ( a ) highlights one putative recombination event in plasmid pB3 and three putative recombination events in plasmid pBP136. The similarity plots of these two plasmids ( b , c ) demonstrate that none of the plasmids included in this study are donors of the recombinant regions in pBP136. Instead, other plasmids from clades that were not previously described were probably involved in these recombination events. Full size image Analysis of genomic signatures Species specificity of a bacterium can be determined by examining its genomic signature (nucleotide patterns found in its DNA) using different approaches. One such approach is the study of genomic compositions of oligomers of different lengths, so-called DNA words [28] . The basis for a particular word frequency rests on a multitude of physicochemical properties, such as base stacking energy, propeller twist angle, bendability, position preference and protein deformability, but is also influenced by the codon usage and GC contents of the DNA [29] . Once a plasmid conjugates to a new host, its signature will ameliorate towards that of the host. By applying recently developed algorithms [30] , [31] , we analysed the genomic signatures in the plasmid backbones to identify putative bacterial hosts. We first created a genomic profile for each of all 1,047 bacterial complete genomic DNA sequences currently available from GenBank. The genomic signatures in the four segments A 1 , A 2 , B and C for each of the 25 plasmids were then matched against these profiles. To test for statistical significance, we started by investigating whether any of the bacterial species within the genus, which contained the best match, had a high probability of being the host. If no significance was found on the genus level, we stepped up one taxonomic level, testing all members in that specific family. If statistical significance was still not detected, this procedure was repeated until we reached the class level. Thus, the P -value indicates whether the signature in a plasmid segment is significantly similar to the signatures of the species in that specific genus, family, order or class ( Fig. 5 ). 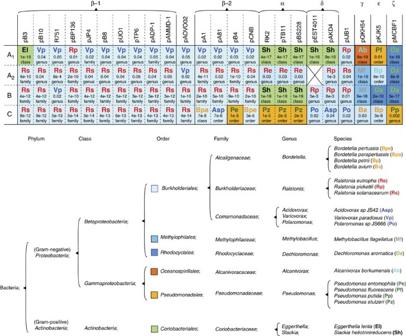Figure 5: Analysis of genomic signatures to identify putative hosts. A signature profile was created according to the word frequency for each of the available 1,047 complete genomic bacterial DNA sequences. Further, segments A1, A2, B and C of each plasmid were tested independently against these profiles. AP-value indicating the statistical significance was also calculated and indicated for each best match together with the taxonomic level for which the significance was achieved. The background colours in the table demonstrate the order that the putative hosts belong to, and the specific host species are denoted as colour-coded abbreviations. Figure 5: Analysis of genomic signatures to identify putative hosts. A signature profile was created according to the word frequency for each of the available 1,047 complete genomic bacterial DNA sequences. Further, segments A 1 , A 2 , B and C of each plasmid were tested independently against these profiles. A P -value indicating the statistical significance was also calculated and indicated for each best match together with the taxonomic level for which the significance was achieved. The background colours in the table demonstrate the order that the putative hosts belong to, and the specific host species are denoted as colour-coded abbreviations. Full size image The majority of the plasmids presented genomic signatures that were most similar to those of species within the phylum Proteobacteria ( Fig. 5 ). Most of these matches were also statistically significant already on the genus or family level. Interestingly, all plasmids had at least two regions with signatures matching species from at least different orders, supporting recombination. In addition, although only statistical significant at the class level, the A 1 segment in plasmid pB3 and all plasmids from the α- and δ-clades, as well as the B-segment in the plasmids from the α-clade, presented a genomic signature most similar to that of species from the Coriobacteriales order of the distantly related Gram-positive phylum Actinobacteria . To further demonstrate recombination, a statistical test for a cross-region comparison was also performed. In this test, only the best match for a specific segment was compared with the best match for the other segments in that plasmid. The results demonstrate statistically different signatures between all segments that had a best hit on the genus or family level in the above test, which further supports recombination between plasmids from different hosts. We analysed the complete backbone genomes of 25 IncP-1 plasmids and demonstrated a divergence into seven distinct phylogenetic clades, that recombination is a common feature of the plasmid backbone evolution, and an adaptation to different hosts. Evolutionary studies of IncP-1 plasmids are often based on gains and losses of transposons and other MGEs [20] , [21] , [22] . In particular, the lack of inserted elements was considered to be a sign of ancestry, as in plasmid pBP136, which has been suggested to represent the ancient ancestor of all IncP-1 β plasmids [22] . However, as MGE are found among plasmids in all described clades, the absence of these may be a poor indicator of ancestry of the IncP-1 group. On the other hand, we demonstrate that plasmid pBP136 is likely to be a recombinant involved in recent recombination events, including parental plasmids from the β-1 subclade and a hitherto unknown clade ( Fig. 4 ). An alternative view would thus be that pBP136 is a result of a β-1 subclade plasmid that has recombined, and exchanged regions, with an ancestral plasmid lacking insertions. Whether there exist such plasmids without insertions or whether insertions can be entirely excised is not yet clear. In any case, frequent insertions and deletions of MGE indicate the recent evolution of plasmids, but the older trajectory of plasmid macroevolution must, as here, be based on events such as the mutation, speciation and recombination of the backbone core regions [32] . All investigated conjugative plasmids, including IncP-1 plasmids, contain at least one entry exclusion gene [33] , which prohibits other plasmids in the same incompatibility family from conjugating to that cell. This exclusion system is believed to confer an evolutionary advantage to the plasmid as it frees the plasmid from competition at segregation during cell division, and protects the plasmid-bearing cell from too many conjugation events [33] , [34] . Laboratory experiments suggest that surface exclusion systems in F-plasmids reduce the conjugation rate 100–300 times, and in IncP-1 plasmids this reduction is 10–15 times [7] , [33] . As our results indicate frequent recombination of IncP-1 plasmids, which requires the presence of two plasmids in one cell, the experimental results indicating that surface exclusion is leaky are supported by this retrospective study. Furthermore, an early study indicates that different IncP-1 plasmids can coexist in one cell for at least 50 generations [35] , which may allow time for recombination. Recombination can function as a powerful and essential driving force of evolution by deleting deleterious mutations [36] , collecting beneficial mutations [37] and increasing the rate of adaptation [38] , [39] . It is tempting to speculate that there is an optimal balance between saving the plasmid from competition by incompatible plasmids and, on the other hand, allowing sporadic mobility and recombination with plasmids evolved in other host bacteria. The three backbone regions in pBP136, identified in the similarity plots, did not present a close similarity to any of the other plasmids included in this study ( Fig. 4 ). A BLAST search, which did not find any sequences with a high similarity with these three regions, suggests that previously undescribed IncP-1 plasmid clades exist. It is therefore likely that we have yet seen only a fraction of the IncP-1 plasmid diversity. No correlation between clade identity and the geographic location of the plasmids was detected by simply comparing isolation site with clade identity. For example, the plasmids of the β-1 subclade were isolated from a hospital (London, UK), a wastewater treatment plant (Braunschweig, Germany), a herbicide spill (Minnesota, USA), industrial sewage (Japan), a mercury-contaminated river (Kazakhstan), Australia and a hospital (Japan) [40] . However, in addition to this apparent worldwide spread, our DNA signature analysis indicates historic isolation of IncP-1 plasmids in specific host bacteria ( Fig. 5 ). Genomic signatures are species specific and likely formed by host replication and repair mechanisms [31] , [41] , [42] , [43] , but may also be affected by environmental factors [44] . Given sufficient residence time, plasmid signatures ameliorate towards that of the chromosome [14] , [28] , [42] . We analysed the putative plasmid–host history by using newly developed algorithms based on DNA words of five nucleotides, which were demonstrated to be superior to G+C or dinucleotide signals for classifying a sequence according to its origin [30] , [31] . The suggested hosts ( Fig. 5 ) are within groups that are known to harbour IncP-1 plasmids [7] . All plasmids, except pMCBF1, had at least one segment with a genomic signature most similar to those of the Burkholderiales order of the Betaproteobacteria class ( Fig. 5 ), signifying the importance of this group as a natural host for IncP-1 plasmids [14] , [41] . The finding that all plasmids had segments that clustered with different hosts was also supported by the cross-region analysis, which further supports recombination. Thus, IncP-1 plasmids are recombinants containing regions in their backbones descending from parental plasmids, which have evolved in different hosts and/or under different selection pressures for sufficient time for these unique genomic signatures to evolve. It is noteworthy that with some exceptions the suggested hosts of each segment A 1 , A 2 , B and C are similar for most members within each clade, indicating that recombination happened early in the clade history and that amelioration towards a common DNA signature is slow. In most cases, the best signature match of a segment was statistically significant on the genus or family level, indicating specific adaptation to a host within that genus or family ( Fig. 5 ). On the other hand, in some examples, the signature of the best match was statistically significant only on the order or class level. The cross-region analysis was also unable to demonstrate a statistically significant difference for these regions. Part of the explanation for this low statistical significance might be that the latter regions have resided in several different hosts and have acquired a mixture of signatures. Further development of bioinformatics tools to analyse mixtures of signatures may provide interesting information about the host history of these plasmids that show low statistically significant match to one specific host. Overall, mean plasmid dinucleotide [41] and trinucleotide signatures [14] were used to suggest plasmid hosts. The latter study showed that the evolutionary host range of the IncP-1 plasmids was broader than the narrow host range of the IncF and IncI plasmids. The hosts suggested in this study, for at least one of the segments in each plasmid, were often close to one of the top five host matches suggested for the overall, whole plasmid analyses by Suzuki et al . [14] . However, in this study we also demonstrate the significance of homologous recombination in the evolution of IncP-1 plasmids. Segment-wise analyses demonstrated that the combination of a broad host range and recombination leads to the emergence of recombinant IncP-1 backbones that contain segments of significantly different host origins. For example, for six plasmids, the A 1 and B segment signatures showed a similarity to bacteria within Gram-positive Actinobacteria ( Fig. 5 ). Interestingly, a recent report showed that the IncP-1 plasmid pKJK5 can transfer to the Gram-positive Arthrobacter sp. strain 108 (also class Actinobacteria ) in soil rhizosphere experiments; this Gram-positive bacterium was in fact the most frequent pKJK5 transconjugant [11] . The manner in which conjugation was detected showed that the plasmid entered the Gram-positive cell and expressed its fluorescence gfp marker gene, but the independent replication of the IncP-1 plasmids was not assessed. It cannot be excluded that IncP-1 plasmids were incorporated into the Gram-positive chromosome and ameliorated, and later recombined to contribute to the present plasmids. Haines et al . [45] recently demonstrated that the IncP-1α plasmid RK2 has a mean G+C content of the backbone of 66.6 mol%, whereas the mean G+C content of pQKH54 (IncP-1γ) is only 56.6 mol%, and suggested that pQKH54 has resided in a host species with a lower G+C content than that of RK2. The mean G+C content for our suggested hosts for RK2 is 63% whereas the mean G+C for the pQKH54 hosts is 57%, which fits well with the plasmid G+C. Moreover, the pKJK5 backbone genes had a 6.3% lower G+C ratio than that of R751, and these two plasmids were also suggested to have had different host histories [19] . The mean G+C content of our suggested hosts of pKJK5 and R751 is 60 and 65%, respectively. Thus, earlier speculations on plasmid relationships based on G+C content [19] , [45] can be substantiated by the DNA signature analysis, which has more predictive power than the G+C content and we can now point to possible hosts. Perhaps the most important aspects of the evolution and adaptation of the IncP-1 backbone to its different bacterial hosts are the role of these plasmids in HGT and transportation of AB R genes [7] , [40] , [46] , which has major implications for the treatment of human pathogens. Several studies have demonstrated that IncP-1 plasmids can spread to [47] , [48] and be maintained in [40] , [49] many different bacteria. Our DNA signature analysis demonstrates that the IncP-1 plasmids have been isolated in, and adapted to, different hosts and/or the specific environments the host cells experienced over evolutionary time scales, implying a plasmid/host coevolution. Although surface exclusion has been known to be leaky [33] and incompatibility does not immediately segregate two plasmids [35] , the extent of direct contact between plasmids in the IncP family is unclear. The frequent pattern of recombination presented here indicates that interactions between IncP-1 plasmid backbones could be direct and not limited to interactions with a third-party MGE. This might be one explanation of the high AB R mobility in the IncP-1 family, strongly supporting the suggestion of Schlüter et al . [7] that IncP-1 plasmids may be viewed as one of the most potent vehicles for the spread and accumulation of multiantibiotic resistance within and between different bacterial communities. Bacterial strains and plasmids and growth conditions Pseudomonas putida UWC1 containing the previously exogenous isolated plasmids pMCBF1 and pMCBF6 (ref. 25 ) were grown overnight at 26 °C in Luria-Bertani medium [50] with 10 g of added NaCl l −1 and supplemented with 17 mg l −1 of HgCl 2 . Escherichia coli were grown overnight at 37 °C in the same medium but supplemented with 50 mg l −1 of ampicillin. Molecular techniques Plasmid DNA was obtained using QIAGEN MIDI preps, according to the manufacturer's recommendations (QIAGEN). Shearing of DNA to create a plasmid library was carried out by sonication for 30 s (Branson 1510 sonicator). Sticky ends were filled with Klenow fragments according to the manufacturer's recommendations (MBI Fermenta). Sheared plasmid DNA was subcloned into the Sma I site of pBluescript II SK+ (Stratagene) by blunt-end ligation, and transformed by heat shock (42 °C, 2 min 30 s) into E. coli XL-1 Blue (Stratagene). Transformants were picked by blue–white selection; plasmid vectors were isolated and screened for inserts by cutting with restriction enzymes, and analysed on standard agarose gels. Vectors with positive inserts were used as templates in sequencing reactions. Sequencing The DNA sequences from the inserts were obtained by using M13 forward and reverse primers from the pBluescript II SK+ and the ABI BigDye Terminator Cycle Sequencing kit (Applied Biosystems). Sequencing was carried out at KI Seq, CGR Sweden, on an ABI 373 automated DNA sequencer (Perkin-Elmer Applied Biosystems). DNA sequences were compiled using Contig Express from the Vector NTI Suite 6.0 (Informax). To close gaps in the sequence, internal custom primers (Invitrogen) were designed. To close gaps and confirm the sequence of the two plasmids, pMCBF1 and pMCBF6 were also sequenced by MWG Biotech AG (Ebersberg; www.mwg-biotech.com ) in a 'publication quality' DNA sequencing project, as described by MWG (both strands sequenced and a final data accuracy of >99.995%). Sequences of pMCBF1 and pMCBF6 were deposited in GenBank; Nucleotide Core #(accession AY950444 and EF107516 ). DNA and AA sequence analysis DNA and AA sequences were aligned by using ClustalW included in the BioX program. Genetic distances were calculated using the protdist program included in the phylip package (phylip 3.66), using the Jones–Taylor–Thornton matrix. Gap regions were not eliminated before this analysis as the program itself drops those regions in affected comparisons. All gap regions were, however, removed from the DNA sequence alignment before the phylogenetic analysis. Phylogenetic network analysis and the φ -statistics were carried out using the SplitsTree program [51] . The splits network (neighbour net) was constructed using the uncorrected P character transformation, which computes the proportion of positions at which two sequences differ, and the bootstrap values were derived from 1,000 bootstrap replicates. The SimPlot and Bootscan analyses were performed by using the SimPlot program [52] , with a window size of 200 and 20 bp steps. All analyses of genomic signatures were based on single intact genomic segments (that is, without alignment and truncation of gap regions). The analysis was carried out by using the program PSTk-Classifier [30] , [31] , with a fixed-order Markov model of order 4 (that is, using a word size of five nucleotides). Profiles were first constructed for each of all 1,047 bacterial complete genome sequences currently available from GenBank. All four segments A 1 , A 2 , B and C in each of the 25 analysed plasmids were then separately matched against these profiles. The Markov classifier determines a score for a bacterium to be the host for a given plasmid. In this way, we can rank various putative host bacteria for a given plasmid. We apply statistical techniques for assessing confidence in our predictions that the top-ranked candidate is the most likely host bacterium: First, we form a list A of the bacteria that are within 5% of the top score. Next, we form a list B of the top-ranked candidate and its closely related neighbours in the Entrez taxonomy database ( http://www.ncbi.nlm.nih.gov/taxonomy ). For this, we traverse the taxonomy up a fixed number of levels and collect all the bacteria that appear below that level. Next we remove from A, those bacteria that also appear in B. Now, our question can be precisely reformulated as follows: Is there a significant difference in scores between the putative hosts in the lists A and B? The null hypothesis is that there is no significant difference, the alternative hypothesis is that there are significantly higher scores in list B. Note that this kind of analysis does not apply to a single putative host but to distinguish two sets of potential hosts. This is required to gain statistical power. In particular, it would assign significance to one taxonomically closely related group of bacteria as being the host as against all the others. We start our analysis on the genus level; that is, we analyse whether the best match is significantly different from the top 5% matches to host bacterial species outside the genus to which the best match belong. If no statistical significance was achieved on the genus level, we moved up one level at a time until the class level was reached. We applied the Mann–Whitney test [53] , a powerful non-parametric statistical test to identify whether two samples of observations have equally large values. It computes a test statistic based on the ranks of the elements in a joint series constructed from the two series. The Mann–Whitney test yields a P -value corresponding to observing a result as extreme as observed series under the null hypothesis. There are several reasons to prefer the Mann–Whitney test in our application to other well-known tests, such as the Student's t -test: First, it is non-parametric, so it does not assume a fixed underlying distribution such as the Normal distribution, which parametric tests such as the Student's t -test do. It is also tailored for ordinal values; that is, the important aspect is the relative order of the data, not their absolute values. This is precisely what we are interested in: the ranks of various bacteria as putative hosts. Furthermore, it is more robust to outliers and hence less likely to assign spurious significance to such data. Finally, it is significantly more efficient than the Student's t -test, especially when the underlying distribution is far away from normal. Another question of interest is whether homologous recombination has created plasmids containing genomic segments, which have evolved in, and adapted to, different host bacterial species. As a complement to the test described above, we performed a cross-region comparison. We compare the best match obtained for each region, and its related neighbours in the hierarchy, against how it compares against the other regions. The null hypothesis is that two regions in a plasmid have evolved in the same host. The alternative hypothesis is that different regions have evolved in different hosts. This test is similar to the test described above with the difference that here we test the best matches against each other irrespective of the top 5% matches. Accession codes: Sequences of pMCBF1 and pMCBF6 have been deposited in GenBank's Nucleotide Core under accession codes AY950444 and EF107516 . How to cite this article: Norberg, P. et al . The IncP-1 plasmid backbone adapts to different host bacterial species and evolves through homologous recombination. Nat. Commun. 2:268 doi: 10.1038/ncomms1267 (2011).